Mycobacterium tuberculosisis extraordinarily sensitive to killing by a vitamin C-induced Fenton reaction Drugs that kill tuberculosis more quickly could shorten chemotherapy significantly. In Escherichia coli , a common mechanism of cell death by bactericidal antibiotics involves the generation of highly reactive hydroxyl radicals via the Fenton reaction. Here we show that vitamin C, a compound known to drive the Fenton reaction, sterilizes cultures of drug-susceptible and drug-resistant Mycobacterium tuberculosis , the causative agent of tuberculosis. While M. tuberculosis is highly susceptible to killing by vitamin C, other Gram-positive and Gram-negative pathogens are not. The bactericidal activity of vitamin C against M. tuberculosis is dependent on high ferrous ion levels and reactive oxygen species production, and causes a pleiotropic effect affecting several biological processes. This study enlightens the possible benefits of adding vitamin C to an anti-tuberculosis regimen and suggests that the development of drugs that generate high oxidative burst could be of great use in tuberculosis treatment. Tuberculosis (TB), a disease caused by the bacillus M. tuberculosis , shares with HIV and malaria the distinction of being one of the deadliest infectious diseases of our time. The World Health Organization estimates that one-third of the world’s population is infected with M. tuberculosis . Chemotherapy, the cornerstone of TB control efforts, is compromised by the emergence of M. tuberculosis strains resistant to several, if not all, drugs available to treat the disease. The development of drug-resistant infections in TB patients is often associated with failure to complete the lengthy chemotherapy. Drug-susceptible TB is treated with isoniazid (INH), rifampicin (RIF), pyrazinamide and ethambutol for 2 months followed by 4 months of INH and RIF, while treatment of multidrug-resistant (MDR) TB can require up to 2 years of chemotherapy with possible damaging side effects. Drugs that kill M. tuberculosis more quickly while also preventing the development of drug resistance could shorten chemotherapy significantly. In the TB pharmacopeia, the first-line drugs INH and RIF are bactericidal, killing 99 to 99.9% of M. tuberculosis cells in vitro within 4 to 7 days. Unfortunately, resistance emerges very rapidly, both in vitro and in vivo [1] , [2] , [3] . In Gram-positive and Gram-negative bacteria, a common mechanism of killing by bactericidal drugs, regardless of their target, involves the generation of hydroxyl radicals by the Fenton reaction [4] (although this mechanism was recently disputed [5] , [6] ) or by protein mistranslation and stress–response two-component system activation [7] . Hydroxyl radicals induce cell death via DNA damage, which is due in part to the oxidation of the guanine nucleotide pool [8] . Hydroxyl radicals can be produced by the combination of the Haber–Weiss cycle [9] and the Fenton reaction [10] . In these reactions, ferrous ion reacts with oxygen to produce superoxide ( 1 ), which by dismutation leads to hydrogen peroxide formation ( 2 ). Hydrogen peroxide then reacts with ferrous ions to form hydroxyl radicals via the Fenton reaction ( 3 ). In the presence of reductants, ferrous ions are produced by reduction of ferric ions. One reductant known to drive the Fenton reaction is vitamin C (VC) (ascorbic acid) [11] . VC is an essential nutrient for some mammals and has potent antioxidant properties. The addition of VC to the human diet has led to the elimination of scurvy [12] and some improvement in the treatment of viral and bacterial infections, cardiovascular diseases, cancer, gout and cataracts [13] , [14] , [15] . Conflicting reports have suggested either beneficial or no effect of VC in the treatment of TB [16] . In the 1930s, McConkey and Smith showed that in guinea pigs, fed with tuberculous sputum and tomato juice simultaneously, only 6% developed intestinal TB, while 70% of the control group, which did not receive any VC supplement, developed ulcerative intestinal TB [17] . A few years later, Pichat and Reveilleau demonstrated that VC could sterilize M. tuberculosis cultures in vitro and postulated that the bactericidal activity could be owing to both VC and its decomposition product(s) [18] , [19] . More recently, VC treatment of M. tuberculosis was found to be bacteriostatic and to induce a dormant drug-tolerant phenotype [20] while another study found a correlation between the high VC content of some medicinal plant extracts and their activity against M. tuberculosis [21] . In this report, we describe the activity of VC against drug-susceptible, MDR- and extensively drug-resistant (XDR) M. tuberculosis . We show that the sterilizing effect of VC on M. tuberculosis in vitro was owing to the presence of high iron concentration, reactive oxygen species (ROS) production and DNA damage. The dramatic killing of drug-susceptible, MDR and XDR M. tuberculosis strains by VC in vitro argues for further studies on the benefits of a high VC diet in TB-treated patients and on the development of bactericidal drugs based on ROS production. High doses of VC sterilize M. tuberculosis cultures in vitro Previous studies on the effect of VC on M. tuberculosis emphasized the fact that high concentrations of VC were necessary to observe any effect [18] . 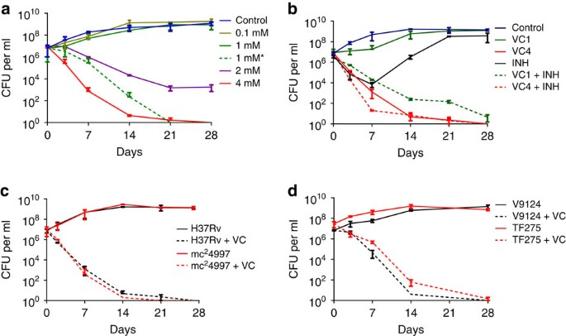Figure 1: VC sterilizes drug-susceptible and drug-resistantM. tuberculosisstrains. (a)M. tuberculosisH37Rv cultures grown to an OD600 nmof≈0.75 were diluted 1/20 and treated with increasing amounts of VC (from 0.1–4 mM). 1 mM* represents an experiment where 1 mM of VC was added to the culture daily for the first 4 days of treatment. (b)M. tuberculosisH37Rv was treated with INH (7 μM, 20 × MIC), VC (1 or 4 mM) and a combination of INH and VC (1 and 4 mM). (c) mc24997, a RIF- and INH-resistantM. tuberculosisH37Rv strain, was treated with VC (4 mM). (d) VC (4 mM) was added to a drug-susceptible strain (V9124) and to an extensively drug-resistant strain (TF275) ofM. tuberculosisfrom the Kwa–Zulu–Natal province of South Africa. Growth was followed and CFUs were determined by plating tenfold serial dilutions and incubating the plates at 37 °C for 4 weeks. The experiments were done at least in triplicate and the average with s.d. is plotted. Therefore, we first determined that the minimum inhibitory concentration (MIC) of VC that prevented the growth of M. tuberculosis was 1 mM ( Table 1 ). Killing kinetic curves were then obtained by treating M. tuberculosis H37Rv with different concentrations of VC (from 1/10 MIC to 4 × MIC) and plating for colony-forming units (CFUs) over the course of 4 weeks. A dose–response relationship was observed and a bactericidal activity was obtained at 2 mM ( Fig. 1a ). Strikingly, 4 mM VC sterilized a M. tuberculosis culture in 3 weeks. At the MIC (1 mM), VC had a brief bacteriostatic effect followed by resumption of growth. As VC is rapidly oxidized into dehydroascorbic acid by air, we examined if the limited activity at 1 mM was owing to VC degradation. M. tuberculosis was treated with daily addition of 1 mM VC for the first 4 days. As a result, M. tuberculosis was killed as rapidly with daily addition of 1 mM VC as with one dose of 4 mM at day 0 ( Fig. 1a ). The killing by VC was not owing to acidification of the media as the addition of 4 mM VC to an M. tuberculosis culture did not alter the pH significantly. The activity of VC against M. tuberculosis led us to test whether VC was also active against other Gram-positive and Gram-negative bacteria ( Table 1 ). Interestingly, VC activity against M. tuberculosis was rather specific as the MICs for non-mycobacteria were at least 16 to 32 times higher than against M. tuberculosis. M. tuberculosis was also the most susceptible strain to VC among the mycobacterial strains tested ( Table 1 ). Table 1 MIC of VC against Gram-positive and Gram-negative bacterial species. Full size table Figure 1: VC sterilizes drug-susceptible and drug-resistant M. tuberculosis strains. ( a ) M. tuberculosis H37Rv cultures grown to an OD 600 nm of≈0.75 were diluted 1/20 and treated with increasing amounts of VC (from 0.1–4 mM). 1 mM* represents an experiment where 1 mM of VC was added to the culture daily for the first 4 days of treatment. ( b ) M. tuberculosis H37Rv was treated with INH (7 μM, 20 × MIC), VC (1 or 4 mM) and a combination of INH and VC (1 and 4 mM). ( c ) mc 2 4997, a RIF- and INH-resistant M. tuberculosis H37Rv strain, was treated with VC (4 mM). ( d ) VC (4 mM) was added to a drug-susceptible strain (V9124) and to an extensively drug-resistant strain (TF275) of M. tuberculosis from the Kwa–Zulu–Natal province of South Africa. Growth was followed and CFUs were determined by plating tenfold serial dilutions and incubating the plates at 37 °C for 4 weeks. The experiments were done at least in triplicate and the average with s.d. is plotted. Full size image To compare the effects of VC to the known mycobactericidal drug INH, we treated M. tuberculosis with VC and/or INH ( Fig. 1b ). For the first 4 days of treatment, the kinetics of killing of M. tuberculosis were similar between INH and 4 mM VC. By 10 days, INH-treated M. tuberculosis gave rise to INH-resistant mutants while VC treatment was still bactericidal. We also tested INH and 4 mM VC together, and the combined action was not antagonistic. Interestingly, 1 mM VC in combination with INH also resulted in sterilization of the culture. One of the main impediments to TB control and eradication is the high prevalence of drug-resistant strains. To assess the effect of VC on drug-resistant strains, MDR (mc 2 4997 (ref. 22 )) and XDR (TF275 (ref. 23 )) M. tuberculosis strains were treated with 4 mM VC for 4 weeks. The killing of mc 2 4997 by VC was indistinguishable from that observed for H37Rv ( Fig. 1c ), resulting in more than 100,000-fold decrease in CFUs in 2 weeks. The activity of VC against TF275 was compared with a putatively ancestral drug-susceptible Kwa–Zulu–Natal strain, V9124 (ref. 23 ) ( Fig. 1d ). With both strains, a 100,000-fold or more reduction in CFUs was observed after 2 weeks of VC treatment, although the XDR-TB strain seemed slightly less sensitive to VC. VC increases iron concentrations in M. tuberculosis cultures In order to decipher the mechanisms underlying the killing of M. tuberculosis by VC in vitro , the isolation of VC-resistant mutants of M. tuberculosis was attempted. In three independent experiments, ~10 9 M. tuberculosis cells were plated on Middlebrook 7H10 plates containing 4 mM VC and despite incubating the plates for over 2 months, no spontaneous mutants ever arose. Next, the transcriptional response of M. tuberculosis to VC (4 mM) after 2 days of treatment was examined. 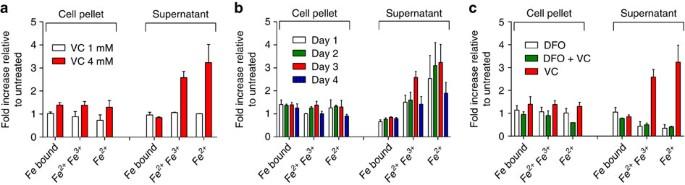Figure 2: VC affects iron concentrations inM. tuberculosis. Iron bound to proteins, total free iron (ferric+ferrous) and free ferrous ion concentrations were measured as described in Methods. Iron concentrations are given relative to untreated.M. tuberculosismc26230 treated with (a) 1 mM or 4 mM VC for 3 days, (b) VC (4 mM) for 1, 2, 3 or 4 days, (c) DFO (100 mg l−1, 152 μM), VC (4 mM) or a combination of both for 3 days. The experiments were done in triplicate and the average with s.d. is plotted. The upregulated genes in VC-treated samples were involved in lipid biosynthesis and intermediary metabolisms such as amino acid, cofactor and carbohydrate biosyntheses and degradation ( Table 2 ). Among the most highly upregulated genes were those encoding enzymes containing divalent cations in their active sites, and this was hypothesized as the displacement of divalent cations by excess iron. This interpretation was supported by the finding that the most downregulated gene, mbtD , is involved in biosynthesis of the siderophore mycobactin ( Table 2 ). When M. tuberculosis is grown in the presence of high concentrations of iron, the levels of mycobactin have been shown to decrease and the mycobactin biosynthesis genes are repressed [24] . There is a duality to the effects of VC: it acts either as an antioxidant or as a pro-oxidant [25] . As a pro-oxidant, VC can drive the Fenton reaction by reducing ferric ions to ferrous ions [11] . Most iron within the cell is bound within porphyrins, and proteins as ferric ions are very sparingly soluble and ferrous ions are very reactive. To examine the role of iron concentration in VC bactericidal activity, the concentrations of bound iron and reduced and oxidized free iron were measured in M. tuberculosis cultures treated with VC. For safety reasons, the experiments were done with mc 2 6230 (H37Rv ΔRD1 Δ panCD ), an M. tuberculosis strain that can be used in a biosafety level 2 laboratory. In VC-treated samples, intracellular free iron levels were increased by 50–75% compared with the untreated cultures after 3 days while extracellular free iron concentrations were nearly fourfold higher than that of the untreated cultures ( Fig. 2a ). This increase in free iron levels was also dose-dependent. With 1 mM VC, which had only a bacteriostatic effect for a brief period, the iron concentrations were similar to the untreated samples ( Fig. 2a ). This large increase in free iron concentrations in the supernatant could also be correlated with a change in supernatant colour in M. tuberculosis treated with VC. Similar to what Pichat and Reveilleau described [18] , we observed that M. tuberculosis cultures treated with VC acquired an orange colour after 24 h. The colouration intensified in the first few days of treatment and then persisted for the duration of treatment. As the colouration of the supernatant appeared within 24 h, iron concentrations were determined over the first 4 days of treatment ( Fig. 2b ). Even at day 1, an increase in free iron content in both the cell pellet and the supernatant was observed, which peaked at day 3. Table 2 Transcriptional profile of VC-treated M. tuberculosis reveals a possible displacement of divalent cations. Full size table Figure 2: VC affects iron concentrations in M. tuberculosis . Iron bound to proteins, total free iron (ferric+ferrous) and free ferrous ion concentrations were measured as described in Methods. Iron concentrations are given relative to untreated. M. tuberculosis mc 2 6230 treated with ( a ) 1 mM or 4 mM VC for 3 days, ( b ) VC (4 mM) for 1, 2, 3 or 4 days, ( c ) DFO (100 mg l −1 , 152 μM), VC (4 mM) or a combination of both for 3 days. The experiments were done in triplicate and the average with s.d. is plotted. Full size image To test whether this increased level in iron correlated with the bactericidal activity of VC, M. tuberculosis H37Rv was treated with VC in the presence of the iron chelator deferoxamine (DFO). M. tuberculosis was first grown with increased concentrations of DFO (from 50–500 mg l −1 ) to determine the highest concentration of DFO that could be used without impairing the growth of M. tuberculosis . A concentration of 100 mg l −1 of DFO had minimal effect on the growth and was therefore selected. When DFO was added to M. tuberculosis H37Rv, VC became bacteriostatic ( Fig. 3a ) and a reduction of 55 and 90% in free ferrous iron was observed in cell pellet and supernatant, respectively, compared with untreated ( Fig. 2c ). 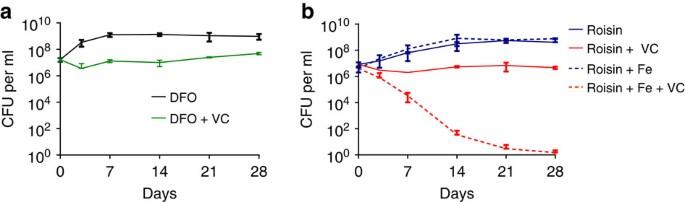Figure 3: The effect of VC is dependent on iron concentration. (a) The iron scavenger DFO inhibits the bactericidal activity of VC againstM. tuberculosisH37Rv.M. tuberculosisH37Rv cultures were grown to an OD600 nmof ≈0.7, diluted 1/20 and treated with with DFO (100 mg l−1, 152 μM) and with or without 4 mM VC. Growth was followed by plating for CFUs over time. (b) The growth ofM. tuberculosisin Roisin medium with and without additional ferric ion (Fe, ferric ammonium citrate (0.04 g l−1)) and treated or not with 4 mM VC was followed by plating for CFUs over time. The experiments were done in triplicate and the average with s.d. is plotted. Figure 3: The effect of VC is dependent on iron concentration. ( a ) The iron scavenger DFO inhibits the bactericidal activity of VC against M. tuberculosis H37Rv. M. tuberculosis H37Rv cultures were grown to an OD 600 nm of ≈0.7, diluted 1/20 and treated with with DFO (100 mg l −1 , 152 μM) and with or without 4 mM VC. Growth was followed by plating for CFUs over time. ( b ) The growth of M. tuberculosis in Roisin medium with and without additional ferric ion (Fe, ferric ammonium citrate (0.04 g l −1 )) and treated or not with 4 mM VC was followed by plating for CFUs over time. The experiments were done in triplicate and the average with s.d. is plotted. Full size image Further confirmation of the role of iron concentration in the bactericidal activity of VC was obtained when VC was found to be bacteriostatic in Roisin’s medium [26] ( Fig. 3b ). Both Middlebrook 7H9 and Roisin’s medium contain ferric ion in their compositions but at different concentrations. Middlebrook 7H9 contains 80 times more ferric ion in the form of ferric ammonium citrate than Roisin. To confirm that the limited availability of ferric ion was responsible for the bacteriostatic effect of VC in Roisin’s medium, ferric ammonium citrate was added to Roisin’s medium in the same amount found in Middlebrook 7H9. In Roisin’s medium supplemented with ferric ammonium citrate, VC regained its sterilizing properties ( Fig. 3b ). VC produces ROS in M. tuberculosis The ability of VC to reduce ferric ions to ferrous ions is well known and is the basis of its pro-oxidant property. The production of ferrous ions leads to the generation of ROS (superoxide, hydrogen peroxide and hydroxyl radicals) via the Harber–Weiss and Fenton reactions, which can result in DNA damage. To test if VC activity against M. tuberculosis could be a consequence of this mechanism, ROS accumulation and DNA damage were measured in M. tuberculosis cultures treated with VC using flow cytometry. Up to threefold increase in total ROS was observed in M. tuberculosis treated with 4 mM VC ( Fig. 4a ). This increase was dependent on the concentration of VC; 0.4 mM VC did not substantially alter total ROS concentration relative to the untreated sample. As a control, the fat-soluble antioxidant vitamin E (VE) was also tested. In contrast to VC, VE had lowered ROS level than the untreated samples after 3 days. To assess the DNA damage potentially caused by ROS accumulation, we measured DNA fragmentation in M. tuberculosis treated with VC or VE using the terminal deoxynucleotidyltransferase-mediated dUTP-biotin nick end labelling (TUNEL) assay ( Fig. 4b ). The percentage of cells with DNA breaks in M. tuberculosis treated with 4 mM VC increased over time to reach 17–25% after 9 days, tenfold higher than in the untreated culture or in the culture treated with VE. 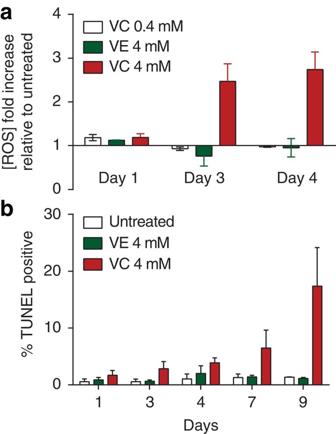Figure 4: VC increases ROS levels and DNA damage inM. tuberculosis. (a)M. tuberculosismc26230 cells treated with low (0.4 mM) or high (4 mM) concentrations of VC or with 4 mM of VE were stained with dihydroethidium. Total ROS concentrations were measured by flow cytometry as described in Methods and followed for 4 days. (b) The percentage of double-stranded DNA breaks were followed over the course of 9 days inM. tuberculosismc26230 treated with VC (4 mM) or VE (4 mM). The experiments were done in triplicate and the average with s.d. is plotted. Figure 4: VC increases ROS levels and DNA damage in M. tuberculosis . ( a ) M. tuberculosis mc 2 6230 cells treated with low (0.4 mM) or high (4 mM) concentrations of VC or with 4 mM of VE were stained with dihydroethidium. Total ROS concentrations were measured by flow cytometry as described in Methods and followed for 4 days. ( b ) The percentage of double-stranded DNA breaks were followed over the course of 9 days in M. tuberculosis mc 2 6230 treated with VC (4 mM) or VE (4 mM). The experiments were done in triplicate and the average with s.d. is plotted. Full size image To further test if this increase in ROS production was one of the mechanisms for the bactericidal activity of VC in M. tuberculosis , cultures were treated with VC in an anaerobic chamber in which the level of oxygen is kept below 0.001%. VC had no effect on M. tuberculosis viability in this condition ( Fig. 5a ). 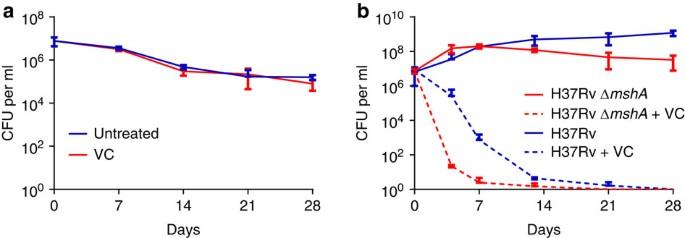Figure 5: VC acts as a pro-oxidant inM. tuberculosis. (a)M. tuberculosismc26230 was grown under aerobic conditions and then shifted to an anaerobic chamber (<0.0001% O2, 5% CO2, 10% H2and 85% N2). After 24 h, the culture was diluted 1/20 with hypoxic media and treated with 4 mM VC. Aliquots were taken at indicated time and plated to determine CFUs. Plates were incubated in an aerobic incubator. (b) The mycothiol-deficient strain H37Rv ΔmshA, grown in Middlebrook 7H9 supplemented with OADC instead of ADS, was treated with 4 mM VC. Growth was followed by plating for CFUs at different times. Both experiments were done in duplicate and the average with s.d. is plotted. Figure 5: VC acts as a pro-oxidant in M. tuberculosis . ( a ) M. tuberculosis mc 2 6230 was grown under aerobic conditions and then shifted to an anaerobic chamber (<0.0001% O 2 , 5% CO 2 , 10% H 2 and 85% N 2 ). After 24 h, the culture was diluted 1/20 with hypoxic media and treated with 4 mM VC. Aliquots were taken at indicated time and plated to determine CFUs. Plates were incubated in an aerobic incubator. ( b ) The mycothiol-deficient strain H37Rv Δ mshA , grown in Middlebrook 7H9 supplemented with OADC instead of ADS, was treated with 4 mM VC. Growth was followed by plating for CFUs at different times. Both experiments were done in duplicate and the average with s.d. is plotted. Full size image Mycothiol-deficient M. tuberculosis is extremely sensitive to VC To examine the cell intrinsic mechanisms of protection from VC-dependent killing, the effect of VC on a M. tuberculosis strain deficient in mycothiol biosynthesis was also assessed. Mycothiol, N -acetyl cysteine glucosamine inositol, is the most abundant low molecular weight thiol in actinomycetes [27] . Its major role is to maintain a reducing environment in the cell; mycothiol mutants have been shown to be hypersensitive to oxidative stress. For example, a M. smegmatis mshA mutant was ten times more sensitive to hydrogen peroxide than the parental strain [28] . M. tuberculosis Δ mshA (ref. 29 ), which does not produce mycothiol [29] , was treated with 4 mM VC for 4 weeks and CFUs were determined ( Fig. 5b ). A rapid 100,000-fold reduction in CFUs was observed after 4 days, much quicker than the wild-type strain. To confirm the hypersusceptibility of the mycothiol-deficient strain to VC, the MIC was determined to be 60-fold lower in the Δ mshA strain than in wild-type M. tuberculosis ( Table 1 ). Complementation of Δ mshA with an integrated copy of M. tuberculosis mshA restored the sensitivity to wild-type level. These results suggest that an oxidative process is part of the VC bactericidal effect. VC affects lipid biosynthesis Lipids are among the most significant targets of oxidative damage. Oxidative damage to membrane and cell wall lipids can impair the essential function of these molecules in the maintenance of homeostasis. The transcriptional analysis revealed that the most upregulated gene in VC-treated M. tuberculosis cultures was psd encoding a phosphatidylserine decarboxylase, which converts phosphatidylserine into phosphatidylethanolamine and is involved in lipid biosynthesis. Interestingly, cell death involving ROS generation was linked to phosphatidylserine translocation on the outer membrane leaflet in E. coli , a phenotype involving psd (ref. 30 ) and described as a marker of the programmed cell death apoptosis [31] . To test the effects of VC on lipids, we performed a pulse-chase experiment where M. tuberculosis was treated with 4 mM VC for 24 h and then labelled with 14 C-acetate for 22 h. Polar lipids ( Fig. 6a ) and fatty acids ( Fig. 6b ) were analysed by thin-layer chromatography (TLC). While all lipid species were present, the total abundance of lipids in VC-treated cells was lower compared with untreated cells. We observed a reduction in the fatty acid levels of VC-treated cells; therefore, we analysed the 14 C-labelled fatty acid samples by high-performance liquid chromatography (HPLC). A general decrease in total fatty acid production in VC-treated samples was observed ( Fig. 6c ), possibly owing to the inhibiting effect of VC on M. tuberculosis growth. The distribution of fatty acids showed a decrease in tetradecanoic (14:0), palmitic/oleic (16:0/18:1) and tuberculostearic (18:0-10Me) acids, with increases in stearic (18:0) and longer-chain fatty acids, consistent with inhibition of the Fatty Acid Synthase type II (ref. 32 ) (FASII) ( Fig. 6d ). Mycobacteria possess two fatty acid synthase systems: the eukaryotic-like fatty acid synthase type I (FASI) and the prokaryotic FASII. M. tuberculosis FASI synthesizes fatty acids in a bimodal pattern (palmitic acid/hexacosanoic acid (26::0)), which are elongated by the FASII system to produce mycolic acids, long-chain (up to 90 carbons) α-alkyl β-hydroxy fatty acids, which are the major constituents of the mycobacterial cell wall. 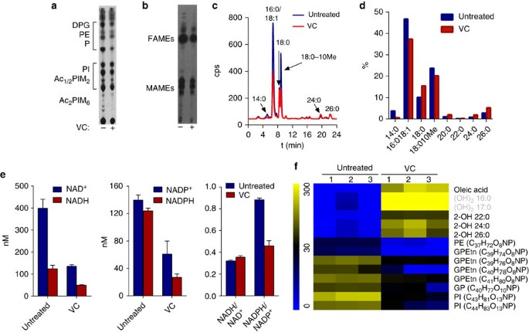Figure 6: VC affects mycobacterial lipids. (a) Polar lipid analysis ofM. tuberculosisH37Rv treated or not with VC (4 mM) for 24 h followed by labelling with14C-acetate for 22 h. Lipids were extracted and analysed on TLC as described in Methods. The same amount of cpm was spotted for each sample. The elution solvent used was CHCl3/MeOH/H2O (10/5/1; v/v/v). DPG, diphosphatidylglycerol; PE, phosphatidylethanolamine; P, unknown phospholipids; PI, phosphatidylinositol; Ac1/2PIM2, mono- and diacyl-phosphatidylinositol dimannosides; Ac2PIM6, phosphatidylinositol hexamannosides (based on ref.48). (b)M. tuberculosisH37Rv was treated with VC (4 mM) for 24 h and then labelled with14C-acetate for 22 h. Fatty acid methyl esters (FAMEs) and mycolic acid methyl esters (MAMEs) were extracted and analysed by TLC as described in Methods. The same amount of cpm was spotted for each sample. (c) Radiolabelled fatty acids used for TLC (b) were saponified and derivatized to UV-absorbing esters for HPLC analysis as described in Methods. (d) Distribution of fatty acids based on the integration of the signals from the HPLC chromatograms shown in (c) 14:0, myristic acid; 16:0, palmitic acid; 18:1, oleic acid; 18:0, stearic acid; 18:0-10Me, tuberculostearic acid; 20:0, eicosanoic acid; 22:0, behenic acid; 24:0, lignoceric acid; 26:0, hexacosanoic acid. (e) NADH, NAD+, NADPH and NADP+concentrations were measured inM. tuberculosistreated with VC (4 mM) for 3 days, as described in Methods. The experiments were done in triplicate. (f) Heatmap representation of the lipids, the most differentially present in the control samples (M. tuberculosismc26230) versus the samples treated with VC (4 mM) for 3 days based on Waters MarkerLynx and Extended Statistics software analysis. In bold are compounds confirmed with standards, and in grey are hypothetical compounds based onm/zand retention time. The other compounds were identified using public mycobacterial lipid databases. The heatmap represents the average of three independent experiments. Figure 6: VC affects mycobacterial lipids. ( a ) Polar lipid analysis of M. tuberculosis H37Rv treated or not with VC (4 mM) for 24 h followed by labelling with 14 C-acetate for 22 h. Lipids were extracted and analysed on TLC as described in Methods. The same amount of cpm was spotted for each sample. The elution solvent used was CHCl 3 /MeOH/H 2 O (10/5/1; v/v/v). DPG, diphosphatidylglycerol; PE, phosphatidylethanolamine; P, unknown phospholipids; PI, phosphatidylinositol; Ac 1/2 PIM 2 , mono- and diacyl-phosphatidylinositol dimannosides; Ac 2 PIM 6 , phosphatidylinositol hexamannosides (based on ref. 48 ). ( b ) M. tuberculosis H37Rv was treated with VC (4 mM) for 24 h and then labelled with 14 C-acetate for 22 h. Fatty acid methyl esters (FAMEs) and mycolic acid methyl esters (MAMEs) were extracted and analysed by TLC as described in Methods. The same amount of cpm was spotted for each sample. ( c ) Radiolabelled fatty acids used for TLC ( b ) were saponified and derivatized to UV-absorbing esters for HPLC analysis as described in Methods. ( d ) Distribution of fatty acids based on the integration of the signals from the HPLC chromatograms shown in ( c ) 14:0, myristic acid; 16:0, palmitic acid; 18:1, oleic acid; 18:0, stearic acid; 18:0-10Me, tuberculostearic acid; 20:0, eicosanoic acid; 22:0, behenic acid; 24:0, lignoceric acid; 26:0, hexacosanoic acid. ( e ) NADH, NAD + , NADPH and NADP + concentrations were measured in M. tuberculosis treated with VC (4 mM) for 3 days, as described in Methods. The experiments were done in triplicate. ( f ) Heatmap representation of the lipids, the most differentially present in the control samples ( M. tuberculosis mc 2 6230) versus the samples treated with VC (4 mM) for 3 days based on Waters MarkerLynx and Extended Statistics software analysis. In bold are compounds confirmed with standards, and in grey are hypothetical compounds based on m/z and retention time. The other compounds were identified using public mycobacterial lipid databases. The heatmap represents the average of three independent experiments. Full size image As FASI and FASII utilize NADPH and NADH as cofactors, respectively, we tested whether the VC effect on fatty acid biosynthesis was owing to a decrease in cofactor availability. Although all cofactor concentrations were decreased by more than half after 3 days of VC treatment, compared with untreated, the NADH/NAD + ratio stayed unchanged while the NADPH/NADP + ratio was reduced by half in the VC-treated samples owing to a larger decrease in NADPH concentration (−80%, Fig. 6e ), suggesting that FASI might be more affected by VC than FASII. For a more accurate and sensitive analysis, total lipids from M. tuberculosis untreated and treated with VC (4 mM) for 3 days were analysed by ultra-performance liquid chromatography-coupled mass spectrometry (UPLC-MS). Only a few lipids were differentially represented in the untreated compared with the VC-treated samples ( Fig. 6f ), including a series of phospholipids (phosphatidylinositols (PI), phosphatidylethanolamines (PE), glycerophosphatidylethanolamines (GPEtn) and glycerophospholipids (GP)), which were found to be five- to eightfold less abundant in the VC-treated samples. Okuyama et al. showed that palmitic, hexadecenoic, octadecenoic and tuberculostearic acids were the major acids found in mycobacterial phospholipids [33] . Tuberculostearic acid has also been found in the mycobacterial cell wall bound to various lipids, such as glycerolipids [34] or phosphoinositides [35] , [36] . This reduction in phospholipids correlates with the results of the HPLC analysis, which showed a decrease in palmitic and tuberculostearic acids. In contrast, VC treatment of M. tuberculosis resulted in an accumulation of unusual hydroxylated fatty acids, which were absent in the untreated samples. The increase in free oleic acid concentration could be owing to the decrease in tuberculostearic acid seen during the total fatty acid analysis ( Fig. 6c ), as oleic acid is the substrate for tuberculostearic acid biosynthesis. We did not detect tuberculostearic acid by UPLC-MS, suggesting that tuberculostearic acid is not present as a free fatty acid but is most likely used in glycerolipid or phospholipid biosyntheses. The effect of VC on various diseases has been widely described and remains controversial [37] . VC is known to be an antioxidant and a pro-oxidant [25] , [38] . The sterilizing effect of VC on M. tuberculosis cultures is most likely owing to its pro-oxidant activity. In this study, we demonstrated that the ability of VC to sterilize M. tuberculosis cultures results from an increase in ferrous ion concentration leading to ROS production, lipid alterations, redox unbalance and DNA damage ( Fig. 7 ). When added to M. tuberculosis in an environment that lacked oxygen or was depleted for iron, VC lost its sterilization capacity. 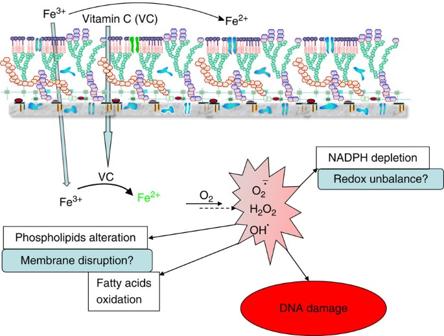Figure 7: Schematic representation of the mechanism of action of VC againstM. tuberculosis. VC entersM. tuberculosiscells and reduces ferric ions to generate ferrous ions that, in presence of oxygen, will produce superoxide, hydrogen peroxide and hydroxyl radicals via the Harber–Weiss and Fenton reactions. The production of these ROS leads to the DNA damage, alteration of lipids and redox balance. Figure 7: Schematic representation of the mechanism of action of VC against M. tuberculosis . VC enters M. tuberculosis cells and reduces ferric ions to generate ferrous ions that, in presence of oxygen, will produce superoxide, hydrogen peroxide and hydroxyl radicals via the Harber–Weiss and Fenton reactions. The production of these ROS leads to the DNA damage, alteration of lipids and redox balance. Full size image Recently, Taneja et al. [20] observed that 10 mM VC induces growth arrest and a ‘dormant drug-tolerant’ phenotype in M. tuberculosis . The authors did not observe a bactericidal activity for VC, even at 10 mM. This difference with our data could be explained by the amount of ferric ion present in their media. Their experiments were carried out in Dubos media, which contains 70% less ferric ions than Middlebrook 7H9. In media with low amounts of iron, it is possible that VC behaves as an antioxidant rather than a pro-oxidant. In their study, the authors also observed that 10 mM VC induced a dormant-like phenotype that rendered M. tuberculosis less susceptible to INH. INH is known to have no activity under non-replicating conditions. Yet in our hands, VC did not reduce the activity of INH. On the contrary, the combination of a sub-lethal concentration of VC (1 mM) with INH resulted in sterilization of M. tuberculosis after 4 weeks ( Fig. 1b ), whereas in vitro treatment of M. tuberculosis with the same amount of INH led to the outgrowth of INH-resistant mutants after 10 days. When INH was combined with VC, no resistant mutants escaped the treatment. This suggests that the addition of sub-inhibitory dose of VC to INH treatment could also reduce the emergence of INH-resistant mutants. We also observed that the sterilizing effect of VC was more substantial in M. tuberculosis strains deficient for mycothiol. Mycothiol is an important reducing agent in M. tuberculosis [27] . Its role is to detoxify and to protect the cells from oxidative damage. In a strain of M. tuberculosis that does not produce mycothiol, the bactericidal effect of VC is increased 60-fold compared with a wild-type strain, resulting in the killing of 10 7 cells in a week. Inhibitors of the enzymes producing mycothiol have been isolated in the hope that they could lead to new drug development [39] , [40] , but a mycothiol-deficient M. tuberculosis strain has no growth defect in vitro and in vivo [29] . Yet, the combination of a mycothiol inhibitor and VC or other pro-oxidant compound could lead to more rapid M. tuberculosis cell death than with most antibiotics used to date. Aside from the generation of ROS species, VC had also an effect on lipid biosynthesis. VC treatment resulted in the generation of free 2-hydroxylated long-chain fatty acids. This is surprising as two comprehensive analyses of total mycobacterial lipids by LC-MS did not reveal the presence of hydroxylated fatty acids in M. tuberculosis [41] , [42] , which we reconfirmed using our own lipid analysis of untreated M. tuberculosis . It is therefore unlikely that these fatty acids are produced by M. tuberculosis . Instead, these fatty acids could be generated by oxidation of 2-alkenoic acid derivatives with hydroxyl radicals from the VC-derived Fenton reaction. In a study by Kondo and Kanai [43] , the authors demonstrated that 2-hydroxyl fatty acids (C16 and C18) were more toxic to mycobacteria than the corresponding saturated fatty acids. This accumulation of 2-hydroxy-fatty acids could therefore lead to a bactericidal event in M. tuberculosis . Furthermore, the reduction in phospholipid content observed in VC-treated M. tuberculosis could affect the mycobacterial cell wall structure and, as a result, M. tuberculosis survival. Interestingly, of several bacteria we tested, M. tuberculosis was the most sensitive to VC. The eight other Gram-positive and Gram-negative bacteria tested were 8- to 32-times more resistant to VC than M. tuberculosis , suggesting that M. tuberculosis could be more sensitive to ROS generation than other bacteria. It could also indicate that against M. tuberculosis , VC has a pleiotropic effect on biological processes such as DNA synthesis, lipid synthesis and redox homeostasis ( Fig. 7 ). This combination of effects might be the reason why VC can sterilize drug-susceptible and drug-resistant M. tuberculosis strains. This is further illustrated by the fact that we were unable to obtain VC-resistant mutants, which is often observed when a drug has multiple targets. This suggests that compounds that generate high levels of ROS could be useful in the development of bactericidal inhibitors of M. tuberculosis , especially if combined with inhibitors of mycothiol biosynthesis. Taneja et al. [20] showed that 2 mM VC added to M. tuberculosis -infected THP-1 cells could arrest the growth of M. tuberculosis , indicating that VC has also some activity against intracellular M. tuberculosis . We believe that the bactericidal activity of VC against drug-susceptible and drug-resistant M. tuberculosis strains supports further studies of the possible combination of TB chemotherapy and a high VC diet in TB patients and offers a new area of research for drug design. Bacterial strains and media M. tuberculosis strains used in this study were obtained from laboratory stocks. Mycobacterial strains were grown in Middlebrook 7H9 medium (Difco, Sparks, MD) supplemented with 10% (v/v) ADS enrichment (50 g albumin, 20 g dextrose, 8.5 g sodium chloride in 1 l water), 0.2% (v/v) glycerol and 0.05% (v/v) tyloxapol. Pantothenate (50 mg l −1 ) was added to the medium to grow M. tuberculosis mc 2 6230. The solid medium used was Middlebrook 7H10 medium (Difco) supplemented with 10% (v/v) OADC enrichment (Difco) and 0.2% (v/v) glycerol. Non-mycobacterial species, except Enterococcus faecalis , were grown in Mueller–Hinton broth (Difco) supplemented with ferric ammonium citrate (0.04 g l −1 ). E. faecalis was grown in Brain Heart Infusion broth (Difco) supplemented with ferric ammonium citrate (0.04 g l −1 ). Cultures were grown at 37 °C while shaking, except for M. marinun , which was grown at 30 °C. All other chemicals were obtained from Sigma or Cayman Chemical unless otherwise noted. Minimum inhibitory concentrations MICs were determined in 2 ml cultures in the appropriate media. The cultures were incubated while shaking for 4 weeks for slow-growing mycobacterial strains and for 2 days for the other bacteria. The MIC was determined as the concentration of VC that prevented growth. Microarray analysis Samples were prepared by adjusting an exponentially growing culture of M. tuberculosis H37Rv to an OD 600 nm ≈0.2 in a 50 ml volume in a 500-ml roller bottle and treating with 4 mM VC. After 2 days of incubation, cells were harvested. RNA was fixed with Qiagen RNA Protect (Qiagen, Germantown, MD). Cells were disrupted by mechanical lysis. RNA was purified with Qiagen RNeasy kit. Contaminating DNA was removed with Ambion TURBO DNA-free. DNA microarrays were provided by the Pathogen Functional Genomics Resource Center (PFGRC) of the J. Craig Venter Institute. Slides were scanned on a GenePix 4000A scanner. TIGR Spotfinder was used to grid and quantitate spots. TIGR MIDAS was used for Lowess normalization, s.d. regularization and in-slide replicate analysis with all quality control flags on and one bad channel tolerance policy set to generous. Results were analysed in MeV with Significance Analysis of Microarrays considered significant at q<0.05 (ref. 44 ). Quantification of iron concentrations Cultures of M. tuberculosis mc 2 6230 were grown to an OD 600 nm ≈0.2. After addition of the appropriate chemicals (VC, DFO), the cultures were incubated for up to 4 days and harvested by centrifugation. The cell pellets were washed twice with ice-cold phosphate-buffered saline (PBS), resuspended in 1 ml 50 mM NaOH with glass beads and lysed using a Fast Prep machine. To quantify bound iron, the lysate (0.1 ml) was mixed with 10 mM HCl (0.1 ml) and 0.1 ml of iron-releasing reagent (1.4 M HCl+4.5% (w/v) aqueous solution of KMnO 4 ; 1/1) and incubated at 60 °C for 2 hours [45] . After cooling, 0.03 ml iron-detection reagent (6.5 mM ferrozine+6.5 mM neocuproine+2.5 M ammonium acetate+1 M ascorbic acid in water) was added and the sample absorbance was read at 550 nm. Total free iron concentration was determined as above without the addition of iron-releasing reagent. Free reduced iron concentration was measured as for the total free iron concentration without the addition of ascorbic acid in the iron-detection reagent. The iron concentrations were determined based on a standard curve obtained with increasing concentrations of ferric chloride and normalized to protein content. Flow cytometry analysis of ROS M. tuberculosis strain mc 2 6230 was grown to OD 600 nm ≈1, diluted 1/5, and treated with VC or VE. Aliquots were taken at the indicated time points and cells were washed twice and stained with dihydroethidium. Cells were immediately used for flow cytometry analysis on a BD FACSCalibur (BD Biosciences, San Jose, CA) with the following instrument settings: forward scatter, E01 log gain; side scatter, 474V log; fluorescence (FL1), 674V log; fluorescence (FL2), 613V log; and threshold value, 52. For each sample, 100,000 events were acquired, and analysis was done by gating intact cells using log phase controls. TUNEL assay Aliquots of mycobacterial cells were removed from M. tuberculosis mc 2 6230 cultures treated with the appropriate compounds and washed once, then fixed in 2% paraformaldehyde for 30 min at room temperature. Cells were centrifuged, permeabilized for 2 min on ice, rewashed and then resuspended in 100 μl of TUNEL reaction mix from the in situ cell death-detection kit (Roche Molecular Biochemicals, Indianapolis, IN). After an incubation period of 1 h at 37 °C in the dark, the reaction mixture was washed once and kept at 4 °C until analysis. Analysis was done by flow cytometry, using the instrument settings described above, by gating intact cells using gamma-irradiated cell-positive controls, and cells incubated with label solution only (no terminal transferase) for negative controls. A total of 100,000 events were acquired per sample. Cells positive for TUNEL staining were quantified as percentages of total gated cells. Polar lipid analysis M. tuberculosis cultures (OD 600 nm =0.2) were treated with VC (4 mM) for 24 h and then labelled with 14 C-acetate (1 μCi ml −1 ) for 22 h. Cell pellets were washed with PBS, autoclaved and extracted with CHCl 3 /MeOH (2/1). The organic phases were dried, resuspended in CHCl 3 /MeOH (2/1; 0.2 ml) and analysed by TLC [46] . Radiolabelled species were detected by autoradiography. The autoradiograms were obtained after exposure at −80 °C for 2 days on X-ray film. Fatty acid analysis M. tuberculosis cultures (OD 600 nm =0.2) were treated with VC (4 mM) for 24 h and then labelled with 14 C-acetate (10 μCi in 10 ml culture) for 22 h. Cell pellets were treated with 20% tetrabutylammonium hydroxide at 100 °C overnight. After cooling, the suspensions were methylated with methyl iodide (0.1 ml) in dichloromethane (2 ml) for 1 h. The organic phase was washed twice and dried [47] . Fatty acids were analysed by TLC (hexane/ethyl acetate; 95/5; 3 elutions). Radiolabelled species were detected by autoradiography as described above. The samples were then saponified with 10% potassium hydroxide in methanol for 2 h at 85 °C and derivatized to UV-absorbing p -bromophenacyl esters using the p -bromophenacyl ester kit from Grace Davison (Deerfield, IL). HPLC analysis of the radiolabelled p -bromophenacyl fatty acid esters was conducted on a Hewlett–Packard model HP1100 equipped with an IN/US β-RAM model 2B flowthrough radioisotope beta-gamma radiation detector (IN/US Systems Inc., Tampa, Fla.). A reverse-phase C18 column (4.6 by 150 mm; 3-mm column diameter; Alltima) was used. The column temperature was set at 45 °C and the wavelength at 260 nm. The mobile phase was acetonitrile and the flow rate was 1 ml min −1 for the first 6 min, followed by a linear increase to 2 ml min −1 in 1 min and then set at 2 ml min −1 for another 17 min. The 14 C-labelled fatty acid esters were detected using the scintillator In-FlowTM ES (IN/US Systems Inc.). The chromatograms’ peaks were identified by comparison with chromatograms of p -bromophenacyl fatty acid ester standards. Cellular concentrations of cofactors M. tuberculosis cultures (OD 600 nm ≈0.15) were treated with VC (4 mM) for 3 days. Fifteen millilitre of each culture was treated with 0.2 N HCl (0.75 ml, NAD + /NADP + extraction) or 0.2 N NaOH (0.75 ml, NADH/NADPH extraction) at 50 °C for 10 min. The samples were neutralized, centrifuged and the supernatants were frozen until ready to use. NADH and NAD + cofactors concentrations were determined spectrophotometrically at 570 nm by measuring the rate of conversion of 3-[4,5-dimethylthiazol-2-yl]-2,5-diphenyltetrazolium bromide (4.2 mM) and phenazine ethosulphate (16.6 mM) by alcohol dehydrogenase (5 units) in the presence of ethanol (20 μl) [44] . NADP + and NADPH concentrations were measured as for NAD + and NADH, using glucose-6-phosphate (4 g l −1 ) instead of ethanol and glucose-6-phosphate dehydrogenase (0.5 unit) instead of alcohol dehydrogenase. Analysis of total lipids by UPLC-MS M. tuberculosis mc 2 6230 (10 ml culture, OD 600 nm ≈0.1) was treated with VC (4 mM) and incubated while shaking for 3 days. The cultures were centrifuged and the cell pellets were washed once with PBS. Lipids were extracted with chloroform/methanol (2/1, v/v; 3 ml) overnight at room temperature while rotating, centrifuged and the supernatants were removed and evaporated to dryness under nitrogen. The lipid residues were dissolved in isopropanol/acetonitrile/water (2:1:1, v/v; 0.75 ml) and analysed by UPLC (Acquity, Waters) coupled with a quadrupole-time of flight mass spectrometer (Synapt G2, Waters). The UPLC column was an ACQUITY BEH C18 Column. The flow rate was 0.5 ml min −1 , the column temperature was set at 55 °C. The mobile phases were: A, acetonitrile/water (60/40) with 0.1% formic acid; B, acetonitrile/isopropanol (10/90) with 0.1% formic acid. The conditions used for the UPLC were: 0 min, 60% A; 2 min, 57% A (curve 6); 2.1 min, 50% A (curve 1); 12 min, 46% A (curve 6); 12.1 min, 30% A (curve 1); 18 min, 1% A (curve 6); 18.1 min, 60% A (curve 6); 20 min, 60% A (curve 1). The MS conditions were: acquisition mode, MS E ; ionization mode, ESI (+/−); capillary voltage, 2 kV (positive), 1 kv (negative); cone voltage, 30 V; desolvation gas flow, 900 l h −1 ; desolvation gas temperature, 550 °C; source temperature, 120 °C; acquisition range, 100–2,000 m/z with a scan time of 0.5 s. Leucine enkephalin (2 ng μl −1 ) was used as lock mass. Data generated from the experiments were processed and analysed by the Waters MarkerLynx software, which integrates, aligns MS data points and converts them into exact mass retention time pairs to build a matrix composed of retention time, exact mass m/z and intensity pairs. Waters Extended statistics software was used to create a two-class OPLS-DA model to identify the mass/retention time pairs that were the most differentially abundant between untreated and VC-treated samples. The noise level was 3% in both positive and negative mode. Ions were identified using published databases ( http://www.lipidmaps.org/tools/ms/LMSD_search_mass_options.php ; http://www.brighamandwomens.org/research/depts/medicine/rheumatology/labs/moody/default.aspx ; http://metlin.scripps.edu/ ). When standards were commercially available, identification was confirmed by comparing retention time accurate mass, and MS/MS data between standards and samples. Accesion codes: The array data have been deposited in the NCBI Gene Expression Omnibus under accession number GSE42293 . How to cite this article: Vilchèze, C. et al. Mycobacterium tuberculosis is extraordinarily sensitive to killing by a vitamin C-induced Fenton reaction. Nat. Commun. 4:1881 doi: 10.1038/ncomms2898 (2013).